Detailed observation of space–charge dynamics using ultracold ion bunches Control of Coulomb expansion in charged particle beams is of critical importance for applications including electron and ion microscopy, injectors for particle accelerators and in ultrafast electron diffraction, where space–charge effects constrain the temporal and spatial imaging resolution. The development of techniques to reverse space–charge-driven expansion, or to observe shock waves and other striking phenomena, have been limited by the masking effect of thermal diffusion. Here we show that ultracold ion bunches extracted from laser-cooled atoms can be used to observe the effects of self-interactions with unprecedented detail. We generate arrays of small closely spaced ion bunches that interact to form complex and surprising patterns. We also show that nanosecond cold ion bunches provide data for analogous ultrafast electron systems, where the dynamics occur on timescales too short for detailed observation. In a surprising twist, slow atoms may underpin progress in high-energy and ultrafast physics. Coulomb interactions can lead to instabilities and emittance growth in charged particle beams, limitting the ultimate performance of electron and ion microscopes [1] , [2] and high-energy particle accelerators [3] . In ultrafast electron diffraction [4] , [5] , [6] , space–charge effects constrain the capacity to obtain diffraction information. For example, in bunches containing just 18 electrons, Coulomb repulsion was shown to increase the bunch duration by 50% and energy spread sevenfold [7] . Coulomb repulsion before [8] and after [9] the specimen thus place an ultimate limit on the ability to extract useful diffraction information. For strongly coupled systems, Coulomb interactions mediate interesting collective effects including the formation of Wigner crystals [10] , self-organization [11] and shock wave phenomena [12] , [13] , [14] . Thus, although the underlying physics of the two-particle Coulomb interaction is simple, the behaviour of beams with complicated spatial and temporal structure can be difficult to predict. Particle trajectory calculations are straightforward for a few particles or even a few million, but become intractable for high-density high-current systems. The development of useful models of self-field effects has been limited by a lack of detailed comparative experimental data where the space–charge and thermal effects are clearly distinguishable. Cold charged particle sources based on near-threshold photoionization of laser-cooled atoms [15] , [16] , [17] , [18] produce electrons and ions with temperatures as low as a few kelvin and millikelvin, respectively, allowing detailed investigation of self-field and strong coupling effects. The ability to arbitrarily shape the initial charged particle distribution [18] enables flexible investigation of the spatial dependence of inter-particle dynamics. The effects of space–charge interactions are enhanced in ion bunches compared with electron bunches. Owing to their high mass, they have comparatively low velocities and hence retain a high charge density following the ionization. The ion temperature is also three to four orders of magnitude lower, allowing distinct measurement of space–charge effects without significant loss of detail due to thermal expansion. During an ionizing laser pulse of time t i in a static electric field, the ion bunch will grow longitudinally as the ions are produced, but the elongation is less than that of an electron bunch created over the same duration due to the larger ion mass. The equivalent-length electron bunch pulse duration t e in the same field is then , where m e,i are the electron and ion mass. The visibility of the space–charge effect is enhanced in ions compared with that in the equivalent-time electron bunches because the ion temperature remains low, with the excess ionization energy predominantly transferred to the photoelectrons. Thus, ion bunches created with ionization pulse durations of a few nanoseconds demonstrate space–charge effects equivalent to those in electron bunches created on picosecond timescales, comparable to the fast electron beams created using cold atom sources [19] , [20] . Pioneering work with cold atom sources has shown evidence of space–charge effects [21] , [22] , and the role of Coulomb interactions in cold ion beams has been studied in detail for continuous-mode low charge density operation [23] , [24] , [25] . In this paper we investigate space–charge effects in arbitrarily shaped nanosecond duration cold ion bunches produced by near-threshold photoionization of laser-cooled atoms. We study in detail a complex ion distribution as an example of the subtle space–charge dynamics that can be observed, in particular the formation of shock wave structures where a halo of cold ions is compressed by the space–charge-driven expansion of a small high-density ion bunch. We observe collective behaviour including high-density caustics and the formation of complex patterns from long-range interaction between small charge bunches. The detail allowed us to systematically test and develop a comprehensive model of the system including self-field effects, illustrating the advantages of observation without thermal diffusion. Generating ultracold ion bunches In our experiments (see Methods), ion bunches were formed by photoionization of an ensemble of laser-cooled rubidium atoms in a magneto-optical trap ( Fig. 1 ). The two-colour ionization process allows ions to be created in an arbitrary charge density profile [18] . The intensity profile of an excitation laser beam (wavelength λ =780 nm, Ω 12 ) was shaped using a reflective phase-shifting spatial light modulator. A second tunable laser (wavelength λ =480 nm, Ω 23 ) was used to couple the excited atoms to a selectable Rydberg state. With the addition of an external static electric field (20–80 kV m −1 ) the atoms are ionized in the region of overlap of the two laser beams. Control of the bunch charge was varied by changing the excitation laser beam power. The ions were accelerated in the static field over a distance of 2.5 cm before drifting 21.5 or 70 cm to a phosphor-coupled microchannel-plate and CCD camera to image the charge density profile of each bunch. 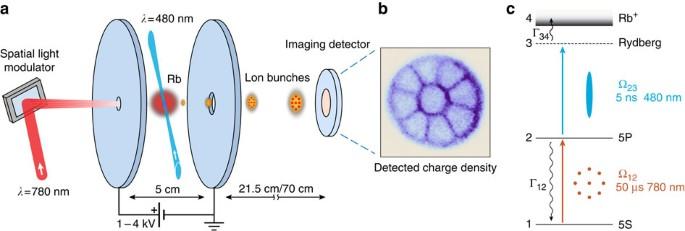Figure 1: Measurement of space–charge dynamics in ultracold ion bunches. (a) Cold rubidium atoms are prepared in a magneto-optical trap. Ions are produced by two-colour near-threshold photoionization. The cold ions are accelerated by a static electric field before drifting 21.5 or 70 cm in a zero-field region to an imaging detector to record their transverse spatial profile. (b) Ion bunch transverse spatial distribution; density shown in false colour. (c) Rubidium energy levels with optical couplings labelled by the Rabi rates Ω, decay rates Γ and schematic transverse laser intensity profiles for relevant states in the two-colour ionization process. Figure 1: Measurement of space–charge dynamics in ultracold ion bunches. ( a ) Cold rubidium atoms are prepared in a magneto-optical trap. Ions are produced by two-colour near-threshold photoionization. The cold ions are accelerated by a static electric field before drifting 21.5 or 70 cm in a zero-field region to an imaging detector to record their transverse spatial profile. ( b ) Ion bunch transverse spatial distribution; density shown in false colour. ( c ) Rubidium energy levels with optical couplings labelled by the Rabi rates Ω, decay rates Γ and schematic transverse laser intensity profiles for relevant states in the two-colour ionization process. Full size image Ring formation At low charge densities, the bunches expand linearly, driven by thermal diffusion. With increasing charge, rather than the simple expansion and loss of detail that might be expected, Coulomb interactions accelerate the growth and induce nonlinear transformation of the bunch structure. 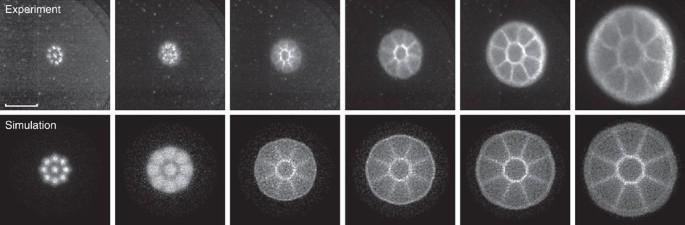Figure 2: Space–charge interactions between ion bunches. Ion beam density profiles imaged 24 cm (7.9 μs) from the source region, for nine closely spaced bunches each of 100 μm diameter. Upper panel: experimentally measured profiles for increasing bunch charge, showing increased expansion and the emergence of high-density regions due to intra-beam space–charge effects. Left to right: shaped excitation laser beam with total power of <1, 70, 210, 340, 640 and 980 μW. Lower panel: simulated bunch structure for ion bunches with spatial profiles calculated with laser profile and powers as used in the experimental images. Total bunch charges of 0 C, 2 fC, 8 fC, 10 fC, 13 fC and 19 fC. The greyscale density profiles are normalized individually to maximize contrast. Scale bar, 5 mm. Figure 2 shows experimentally measured projected ion bunch densities, for nine small closely spaced ion bunches. At low-excitation laser power (low bunch charge; left column) the measured distribution after propagation closely matches the intensity profile of the excitation laser and original bunch shape. Increased laser power and bunch charge induce surprisingly complex structure due to Coulomb interactions within and between the bunches. In particular, we observe the formation of high-density rings and collision boundaries between bunches. Figure 2: Space–charge interactions between ion bunches. Ion beam density profiles imaged 24 cm (7.9 μs) from the source region, for nine closely spaced bunches each of 100 μm diameter. Upper panel: experimentally measured profiles for increasing bunch charge, showing increased expansion and the emergence of high-density regions due to intra-beam space–charge effects. Left to right: shaped excitation laser beam with total power of <1, 70, 210, 340, 640 and 980 μW. Lower panel: simulated bunch structure for ion bunches with spatial profiles calculated with laser profile and powers as used in the experimental images. Total bunch charges of 0 C, 2 fC, 8 fC, 10 fC, 13 fC and 19 fC. The greyscale density profiles are normalized individually to maximize contrast. Scale bar, 5 mm. Full size image The rings are visually similar to those formed by the interplay between self-fields and external focusing elements in electron storage rings [26] , but in our case are found for all high-density initial distributions regardless of beam size and internal profile. The rings are also suggestive of phase–space wave-breaking phenomena, which have been predicted for particle beams [27] , [28] , [29] , and similar to shock-shell formation predicted, but not yet experimentally observed, for Coulomb explosion of strongly coupled plasmas formed from cold ions [13] and in laser-irradiated nanoclusters [30] . We also observe high-density layers at the collision between expanding bunches. These layers have an apparent stickiness or adherence, in that the separate rings do not expand through each other, but compress to form collision boundaries. The compression layers have not been observed in studies of merging electron beams [31] , illustrating the insight available through investigation of space–charge effects with cold and heavy ions. Simulation and modelling The evolution of the ion bunches was simulated using General Particle Tracer [32] , which propagates point particles through the known accelerator field structures and the dynamically evolving self-field. The initial charge distributions were determined from the measured laser spatial profiles by calculation of the atomic excitation. For two-step ionization at a high 480-nm pulse energy, the probability of ionization is proportional to the probability of being in the intermediate 5P state before the 480-nm laser pulse [18] , [24] , [33] , but the usual expectations of saturation for a two-level transition [34] are not applicable since we must include loss via field ionization. Indeed, experimentally, we can infer the number of ions produced from the space–charge-induced bunch expansion ( Fig. 2 ) and we did not observe saturation of ion production even at several hundred times saturation intensity for the 480-nm transition. We developed a four-level model of the excitation and ionization process (see Methods), with field ionization included as a fixed rate loss. The extension accounts for laser-induced transitions from the ground to excited state during the 5-ns ionizing laser pulse, such that the ionization fraction is not limited by the saturated excited-state fraction before the ionization pulse. The spatial charge distribution of the ion bunches was calculated by numerical solution of four-level optical Bloch equations, given the known laser intensity profiles. We included the effects of fluorescence and reabsorption of the 780-nm photons, which lead to the formation of a halo of ions at large distances from the laser intensity maxima. The overall effect for a Gaussian excitation beam is an ion charge distribution that is radially broadened from the laser profile with a long, smoothly decreasing tail at large radius. The experimentally observed high-density rings that surround the ion bunches were reproduced in simulation. 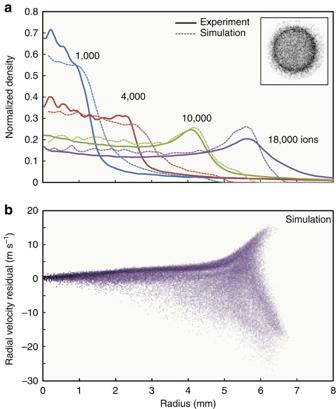Figure 3: Ion bunch profiles. (a) Measured and calculated radial dependence of the ion density. (b) Logarithm of the ion phase–space density, showing two orders of magnitude in density from light to dark, for a single bunch of 18,000 cold ions at propagation distance and time of 70 cm and 10.8 μs, respectively. The formation of a shock front at the outer edge of the bunch is illustrated by the caustic in the phase–space distribution. Inset ofashows typical measured density profile for a single bunch. Figure 3a shows the axially averaged radial distribution calculated for expanding ion bunches of varying charge density. The rings are formed by the dense inner core of ions, expanding rapidly due to Coulomb repulsion, until they interact with cold low-density ions in the halo generated by the reabsorption of fluorescence during the excitation phase. This behaviour is consistent with analytic predictions of the Coulomb explosion of dense nanoclusters irradiated by ultra-intense laser fields on very short timescales, which are studied in the context of laser-triggered nuclear fusion [30] , [35] , [36] , [37] . Figure 3: Ion bunch profiles. ( a ) Measured and calculated radial dependence of the ion density. ( b ) Logarithm of the ion phase–space density, showing two orders of magnitude in density from light to dark, for a single bunch of 18,000 cold ions at propagation distance and time of 70 cm and 10.8 μs, respectively. The formation of a shock front at the outer edge of the bunch is illustrated by the caustic in the phase–space distribution. Inset of a shows typical measured density profile for a single bunch. Full size image Figure 3b shows the simulated phase–space structure of a high-density bunch, in particular showing the large radius and momentum ring that are akin to shock wave formation in strongly interacting media. Modelling of a similar initial distribution of cold ions, in one dimension and without the halo formed by reabsorption of spontaneous emission, has also predicted an expanding shock front [13] , but the formation of high-density boundary layers at the collision of the expanding ion shells has not been previously reported [31] . The negligible thermal diffusion of the ions in our experiments allows direct observation of the shells and high-density boundary layers despite the comparatively low density and long timescales. Simulations of the equivalent-time electron bunches show the same structures forming at very low initial electron temperature, but loss of visibility at a few kelvin, the lowest electron temperatures currently achievable [18] , [20] . Model verification The high-density rings of our ion bunches are formed as the expanding core interacts with a halo of surrounding cold ions produced from reabsorbed spontaneous emission. The link between spontaneous emission and ring structure was tested by varying the duration of spontaneous emission before ionization and measuring the effect on ring density. The spontaneous emission time was determined by the delay between the 780- and 480-nm laser pulses used in the two-step ionization process. The first laser excites atoms to the 5P 3/2 state, which has a natural lifetime of 26 ns. The second laser, with pulse length of 5 ns, excites the 5P atoms to a resonant auto-ionizing state in the static ambient electric field. The fluorescence from the intermediate 5P state can therefore be controlled by varying the delay between the two laser pulses, allowing variation of the density of excited and subsequently ionized atoms in the halo. 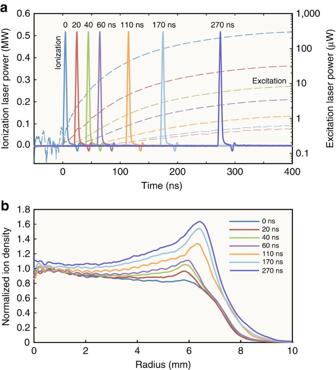Figure 4: Halo formation via fluorescence. Variation in density of halo ions with excitation laser pulse temporal separation. (a) Solid lines (left) and dashed lines (right) show the blue ionization and red excitation laser pulse timing. The excitation laser rise time is limited by the acousto-optical modulator used to modulate the laser beam. (b) Measured ion bunch radial profiles for varying ionization delay, for free-propagation distance of 70 cm. Owing to the slow rise of the excitation laser intensity, the charge density of the beam ‘core’ was kept constant for different timings by adjusting the power of the excitation laser. With a constant core density the expansion rate is approximately constant, but the 5P–5S fluorescence increases with pre-ionization excitation delay, increasing the halo density. Figure 4 shows the variation in visibility of the outer rings in the propagated bunch with changing time between pulses, showing increasing visibility with increased duration of spontaneous emission. Figure 4: Halo formation via fluorescence. Variation in density of halo ions with excitation laser pulse temporal separation. ( a ) Solid lines (left) and dashed lines (right) show the blue ionization and red excitation laser pulse timing. The excitation laser rise time is limited by the acousto-optical modulator used to modulate the laser beam. ( b ) Measured ion bunch radial profiles for varying ionization delay, for free-propagation distance of 70 cm. Owing to the slow rise of the excitation laser intensity, the charge density of the beam ‘core’ was kept constant for different timings by adjusting the power of the excitation laser. With a constant core density the expansion rate is approximately constant, but the 5P–5S fluorescence increases with pre-ionization excitation delay, increasing the halo density. Full size image The evolution of the multi-beamlet ion bunch is shown in an animation ( Supplementary Movie 1 ), where each frame is the calculated charge density profile for one charge bunch, in a plane transverse to the bunch propagation direction. The simulated ion bunch contains nine mini-bunches of 10 4 ions each, plus 2 × 10 4 simulated halo ions, for an accelerating field of 20 kV m −1 over 2.5 cm and free propagation of 14 cm (5 μs). The space–charge-driven bunch expansion and formation of the halo rings and colliding beamlets are readily apparent. Cold atom-charged particle sources are a promising new approach to producing high-brightness beams for applications in ultrafast imaging and high-resolution nanoscale fabrication. Achieving that promise will require detailed understanding of the Coulomb interactions within charge bunches and we have shown here that cold ion bunches can be a powerful tool for investigating such charged particle beam behaviour. The detailed measurements that are possible with cold ions have allowed us to test predictions of complex interactions in high-density charge bunches. Our observations highlight the importance of the initial charge density resulting from the photoionization process and identify the origin of features such as high-density caustics and inter-bunch boundary layers, which indicate nonlinear fields that lead to the emittance growth. The ability to arbitrarily shape the bunches in three dimensions has made it possible to mimic the density distributions for complex and diverse source configurations and probe the associated beam quality degradation related to space–charge effects. The low temperature of cold ion sources, and the scaling of time due to the electron/ion mass ratio, allows precise measurement of previously inaccessible space–charge dynamics relevant to high-density electron bunches used in accelerators and ultrafast electron diffraction imaging. Experimental apparatus and techniques A magneto-optical trap loaded from an effusive oven source and a Zeeman slower [38] was used to collect neutral rubidium-85 atoms at a temperature of 70 μK in a region ~5 mm in diameter, with a peak density of 1.2 × 10 10 cm −3 . The atoms were ionized by two-step, near-threshold photoionization. A λ =780 nm laser beam was used to drive the first-step excitation transition. This beam consisted of two laser frequencies, with 900 μW of power tuned to the 5 2 S 1/2 (F=3)→5 2 P 3/2 (F=4) transition and 100 μW acting as a repumper on the 5 2 S 1/2 (F=2)→5 2 P 3/2 (F=3) transition. The excitation laser beam intensity profile was shaped with a spatial light modulator to control the spatial distribution of the intermediate excited-state atoms in two dimensions. Atoms in the 5P state were then excited to a field-ionizing state, equivalent in energy to an n ≃ 30 Rydberg state in a null field, by a λ =480 nm, 2–6 mJ laser pulse of 5 ns duration focused to a 100 μm × 8 mm (full width at half maximum) ribbon propagated perpendicular to the excitation laser beam, defining the profile of the ions along the direction of ion propagation. The atoms were excited and ionized in a static electric field of 20–80 kV m −1 between a pair of parallel plate electrodes. During and shortly after ionization, heating processes such as disorder-induced heating increase the ion temperature to a few millikelvin [39] . The ion bunches were accelerated over a distance of 2.5 cm, traversed an aperture in the grounded electrode and expanded due to the strong lens effect of the aperture, then drifted in a field-free region for 21.5 ( Fig. 2 ) or 70 cm ( Figs 3 and 4 ) to a phosphor-coupled microchannel plate and the spatial charge density was imaged with a CCD camera. Modelling and simulation To simulate the propagation of the cold ions with space–charge effects included, we first calculated the initial spatial profile of the bunches. The atomic state was described with a four-state density matrix for the electronic ground and intermediate excited states, the resonant self-ionizing state and the final ionized state. The states were coupled by laser fields with position- and time-dependent intensities and by spontaneous decay (see Fig. 1c ). Field ionization was represented by rate Γ 34 , which was determined from calculated near-threshold ionization cross-sections [40] . The evolution of ρ , the density matrix for the four-level atom, is given by where the indices are associated with the atomic levels given in Fig. 1 . The Hamiltonian for the laser–atom interaction is The decay terms are: The optical Bloch equations for the four-level system were derived following standard approaches [34] , [41] and solved numerically for the spatially varying time derivative of the population of the ionized state. The total bunch charge was adjusted to optimize the agreement with the measured density distribution. Particle tracking simulations [32] were used to calculate the evolution of the ion bunches under the influence of the external accelerator fields and internal Coulomb self-fields, as shown in the animation ( Supplementary Movie 1 ). The tracking simulations reveal the time dependence of the bunch evolution, and two-dimensional projections of the particle density can be compared with experimental results as in Fig. 2 . The essential features of the calculated initial bunch profiles produced good qualitative agreement with the observed bunch behaviour. Simulations were performed using a three-dimensional particle mesh method to calculate the self-field, and also by calculating the interactions between all ion pairs. The bunch evolution was identical for the two approaches, showing that for our initial distributions, the evolution was dominated by space–charge effects rather than statistical Coulomb (Boersch) effects, which would not be apparent with the mesh method. The effects of fluorescence and reabsorption of the quasi-continuous excitation beam were included using a first-order single-scattering approximation. Assuming steady-state conditions before the ionizing laser pulse, the excited-state spatial profile without fluorescence ρ 22 ( x ) was calculated from the laser intensity. Excited atoms spontaneously emit photons at the natural decay rate Γ 21 , so the scattered light intensity is assuming isotropic emission, where ℏ ω is the energy per photon and N ( x ) is the atomic number density. The scattered intensity is then added to the laser intensity to calculate the initial conditions of the excited-state profile corrected for reabsorption. Saturation and reabsorption cause broadening of the excited-state profile compared with the excitation laser profile, and the appearance of a halo of excited-state atoms that decrease in density smoothly from the beam core out to long distances. This excitation halo is ionized, becoming responsible for the formation of a density wave at the edge of an exploding ion bunch. How to cite this article: Murphy, D. et al. Detailed observation of space–charge dynamics using ultracold ion bunches. Nat. Commun. 5:4489 doi: 10.1038/ncomms5489 (2014).